Host iron status and iron supplementation mediate susceptibility to erythrocytic stagePlasmodium falciparum Iron deficiency and malaria have similar global distributions, and frequently co-exist in pregnant women and young children. Where both conditions are prevalent, iron supplementation is complicated by observations that iron deficiency anaemia protects against falciparum malaria, and that iron supplements increase susceptibility to clinically significant malaria, but the mechanisms remain obscure. Here, using an in vitro parasite culture system with erythrocytes from iron-deficient and replete human donors, we demonstrate that Plasmodium falciparum infects iron-deficient erythrocytes less efficiently. In addition, owing to merozoite preference for young erythrocytes, iron supplementation of iron-deficient individuals reverses the protective effects of iron deficiency. Our results provide experimental validation of field observations reporting protective effects of iron deficiency and harmful effects of iron administration on human malaria susceptibility. Because recovery from anaemia requires transient reticulocytosis, our findings imply that in malarious regions iron supplementation should be accompanied by effective measures to prevent falciparum malaria. The interactions between falciparum malaria and iron deficiency anaemia (IDA) are complex and bi-directional. Malaria causes acute anaemia by destroying both infected and uninfected red blood cells (RBCs) [1] , whereas persistent sub-clinical infection causes a milder anaemia of infection by blocking iron recycling to the bone marrow [2] . Conversely, once established, IDA protects both pregnant women [3] , [4] , [5] and children [6] , [7] , [8] from malaria. In addition, supplemental iron, given alone or in combination with other micronutrients, predisposes children to malaria [8] , [9] and other serious adverse outcomes [10] . Iron homeostasis has been implicated in regulating liver stage P. falciparum infection; in murine studies, erythrocytic stage malaria infection initiates hepcidin-mediated hepatic hypoferremia, which blocks superinfections by sporozoites from competing plasmodial strains [11] . Mathematical modelling suggests that this can explain the low levels of superinfections in young children [11] , but this mechanism cannot account for observed reductions in the risk of primary malaria infection in children with IDA. It has also been speculated that transient peaks in non-transferrin-bound iron caused by administration of highly absorbable iron supplements [12] could promote intra-erythrocytic parasite growth [13] or bacterial septicemia (a common cause of death in malaria patients [14] , [15] , [16] ) but definitive evidence is absent. As iron deficiency and iron supplementation of iron deficient individuals profoundly alters erythropoiesis, RBC physiology, and RBC population structure, we hypothesized that iron deficiency and iron supplementation directly impact the disease causing erythrocytic stage of P. falciparum infection. In our investigations, we minimize the confounding factors that have complicated prior field studies of the relationship between host iron status, iron supplementation and falciparum malaria by utilizing an in vitro system with freshly isolated RBCs from donors with well-defined, physiologic iron states recruited through our US-based hospital clinic. This approach eliminated the influence of acquired and innate immunity to malaria, haemoglobinopathies and concurrent inflammation. Our study reveals that RBCs from donors with IDA confer malaria protection by impairing P. falciparum invasion and intra-erythrocyte propagation. This protective effect was reversed when donors with IDA received iron supplementation. We go on to show that when iron-deficient RBCs are replaced with iron-replete (IR) RBCs in vitro (as occurs in individuals with IDA following iron supplementation) the susceptibility to P. falciparum infection is increased. These findings support well-described clinical patterns of differential susceptibility to malaria. Taken together, they indicate that therapeutic iron supplementation conspires with host iron status to mediate host RBC susceptibility to malaria infection by altering the dynamic structure of the host’s RBC population. Malaria growth is reduced in RBCs from individuals with IDA To determine the effect of IDA on the growth of erythrocytic stage P. falciparum , we enrolled donors with and without IDA from a non-malaria endemic area through our US-based hospital clinic. 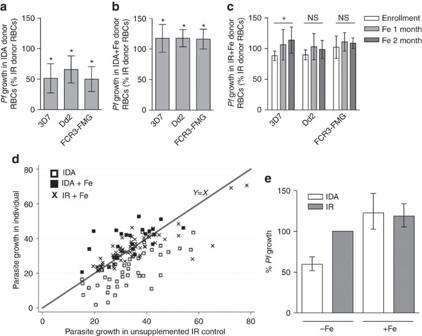Figure 1:P. falciparumgrowth is reduced in iron-deficient RBCs and iron supplementation eliminates growth attenuation. (a–c) Growth experiments with RBCs from IDA donors (n=7), IDA+Fe donors (n=5) and IR+Fe donors (n=4) were performed. Growth rate in RBCs from an IR donor served as the control. Bars represent growth ofP. falciparum(strains 3D7, Dd2 and FCR3-FMG) in indicated RBCs, normalized to growth in RBCs from IR donors (% Pf growth in IR RBC). Error bars represent the s.d. (a) Bars represent growth in RBCs from IDA donors. Significance was determined by two-tailed paired Student’st-test. *P<3E−10as compared withP. falciparumgrowth in RBCs from IR donors. (b) Bars represent growth in RBCs from IDA+Fe donors. Significance was determined by two-tailed paired Student’st-test. *P<0.0003 as compared withP. falciparumgrowth in RBCs from IR donors. (c) Bars represent growth ofP. falciparumin RBCs from IR+Fe donors at enrollment, 1 month and 2 months on iron, normalized to growth in RBCs from IR donors (% Pf growth in IR RBC). Significance was determined by one-way analysis of variance.†P<0.02 for strain 3D7and nonsignificant (n.s.) for strains Dd2 and FCR3-FMG. (d) Mean growth rate ofP. falciparumin RBCs from each individual IDA (□), IR+Fe (x) and IDA+Fe (▪) donor plotted against the growth rate ofP. falciparumin corresponding control RBCs from non-supplemented IR donors. Data were analysed by mixed effects regression. The Y=X line was fit to the growth rates (in RBCs from IR donors). Points below the Y=X line indicate growth rates less than that within RBCs from IR donors. (e) Graphical summary of the mixed effects regression analysis shown ind. Donor and parasite preparation were fitted as crossed random effects. The bars show the estimated parasite growth ofP. falciparumin RBCs from the IDA, IDA+Fe and IR+Fe donors as a percent ofP. falciparumgrowth in RBCs from non-supplemented IR donors. Error bars represent the 95% confidence interval. Donors were classified as IR (haemoglobin (Hgb) >11 g dl −1 , mean corpuscular volume (MCV) >80 fL, ferritin >12 ng ml −1 ) or as IDA (Hgb <11 g dl −1 , MCV <80 fL, ferritin <12 ng ml −1 ) ( Table 1 ). Non-anaemic donors with low-iron stores (Hgb >11 g dl −1 , ferritin <12 ng ml −1 ) were excluded. P. falciparum (strains 3D7, Dd2 and FCR3-FMG) were grown in either RBCs from the IR ( n =10) or IDA ( n =7) donors in up to three consecutive 96 h growth assays ( Supplementary Fig. 1 ). We observed that parasite growth rates were reduced in RBCs from IDA donors as compared with growth in RBCs from IR donors by 48.8% (standard deviation (s.d. )±23.9), 34.3% (s.d.±22.2) and 50.0% (s.d.±20.4) for strains 3D7, Dd2 and FCR3-FMG, respectively ( Fig. 1a ). These findings clearly show that P. falciparum propagation is reduced within RBCs from IDA individuals, but that variability may exist in the degree to which different P. falciparum isolates are affected by IDA. Table 1 Iron parameters and values of study participants. Full size table Figure 1: P. falciparum growth is reduced in iron-deficient RBCs and iron supplementation eliminates growth attenuation. ( a – c ) Growth experiments with RBCs from IDA donors ( n =7), IDA+Fe donors ( n =5) and IR+Fe donors ( n =4) were performed. Growth rate in RBCs from an IR donor served as the control. Bars represent growth of P. falciparum (strains 3D7, Dd2 and FCR3-FMG) in indicated RBCs, normalized to growth in RBCs from IR donors (% Pf growth in IR RBC). Error bars represent the s.d. ( a ) Bars represent growth in RBCs from IDA donors. Significance was determined by two-tailed paired Student’s t -test. * P <3E −10 as compared with P. falciparum growth in RBCs from IR donors. ( b ) Bars represent growth in RBCs from IDA+Fe donors. Significance was determined by two-tailed paired Student’s t -test. * P <0.0003 as compared with P. falciparum growth in RBCs from IR donors. ( c ) Bars represent growth of P. falciparum in RBCs from IR+Fe donors at enrollment, 1 month and 2 months on iron, normalized to growth in RBCs from IR donors (% Pf growth in IR RBC). Significance was determined by one-way analysis of variance. † P <0.02 for strain 3D7and nonsignificant (n.s.) for strains Dd2 and FCR3-FMG. ( d ) Mean growth rate of P. falciparum in RBCs from each individual IDA (□), IR+Fe (x) and IDA+Fe (▪) donor plotted against the growth rate of P. falciparum in corresponding control RBCs from non-supplemented IR donors. Data were analysed by mixed effects regression. The Y=X line was fit to the growth rates (in RBCs from IR donors). Points below the Y=X line indicate growth rates less than that within RBCs from IR donors. ( e ) Graphical summary of the mixed effects regression analysis shown in d . Donor and parasite preparation were fitted as crossed random effects. The bars show the estimated parasite growth of P. falciparum in RBCs from the IDA, IDA+Fe and IR+Fe donors as a percent of P. falciparum growth in RBCs from non-supplemented IR donors. Error bars represent the 95% confidence interval. Full size image Malaria growth is increased in RBCs from iron-supplemented donors Given field evidence that supplementation of children with 12.5 mg of iron (1–1.5 mg kg −1 ) and 50 ng of folic acid may potentiate the risk of malaria [9] , we next investigated the effects of iron supplementation of IDA and IR individuals on in vitro growth of erythrocytic stage P. falciparum. We first collected RBCs from IDA patients who were receiving iron supplementation (IDA+Fe); these individuals met the above criteria for IDA and were receiving either high-dose oral ferrous sulfate (60 mg elemental iron orally three times per day (9–12.6 mg kg −1 )) or intravenous iron (at a dosage determined by their personal physician using the following equation: Dose=0.0442 [desired Hgb—observed Hgb] × LBW+[0.26 × LBW]). IDA+Fe group Hgb values ranged from 6.6 to 9.8 g dL −1 and MCV values ranged from 75 to 98 fL. Additionally reticulocyte counts and red cell distribution width (RDW) were elevated; and average mean corpuscular haemaglobin concentration (MCHC), total iron, and ferritin values were greater than that of the IDA group but still lower than that of the IR group ( Table 1 ). Together, these values are indicative of an erythropoietic response to iron supplements, but not full recovery from IDA. Comparison of the growth rate of P. falciparum (strains 3D7, Dd2 and FCR3-FMG) within RBCs from the IDA+Fe donors to the growth rate of parasites within RBCs from IR donors revealed increases in P. falciparum growth of 17.3% (s.d.±22.7), 17.6% (s.d.±14.0) and 26.3% (s.d.±16.1) for 3D7, Dd2 and FCR3-FMG in RBCs from IDA+Fe donors ( Fig. 1b ). We additionally assessed the effect of iron supplementation of IR individuals on P. falciparum growth. For this study, IR individuals donated blood at enrollment (baseline) and were then prescribed daily oral iron supplementation (325 mg ferrous sulfate). Iron-supplemented IR study participants (IR+Fe) subsequently returned at one and two months following initiation of daily iron supplementation to donate blood. At each donation (enrollment, 1 month and 2 months), the growth rate of P. falciparum (strains 3D7, Dd2 and FCR3-FMG) within RBCs from IR+Fe donors was determined and then compared with the corresponding parasite growth rates within RBCs from a non-supplemented IR donor. Compared with RBCs from IR donors, we observed in RBCs from IR+Fe donors that 1 month of iron supplementation increases of 17.5% (s.d.±16.1), 11.3% (s.d.±15.7) and 6.6% (s.d.±8.1) in growth for 3D7, Dd2 and FCR3-FMG, respectively. There was no change in parasite growth rate in RBCs collected 1 and 2 months after administering iron supplements ( Fig. 1c ). Analyses of Hgb, haematocrit, MCV, MCHC, transferrin saturation, ferritin and reticulocyte count of IR+Fe donors revealed no significant change in their iron status following iron supplementation ( Table 1 ). To comprehensively compare and ultimately quantify the impact of IDA and iron supplementation on the growth of P. falciparum in vitro , we integrated data from all growth experiments and fit a multilevel random effects model to the pooled data ( Fig. 1d ). The outputs of this analysis were growth rates of any parasite strain in experimental RBCs plotted against the growth rate in IR RBC controls. Values were adjusted for variation between study participants, day-to-day differences in parasite preparations and differences in P. falciparum strain growth rates. The Y=X line was fit to the growth rate of P. falciparum in RBCs from IR donors. Data above the Y=X line indicate growth rates greater than that of parasite growth in RBCs from IR donors and data below the Y=X line indicate growth rates lower than that of parasite growth RBCs from IR donors. Based on this analysis, we estimate that compared with IR RBCs, P. falciparum growth is reduced (59.8% (95% confidence interval (CI)=51.9–68.8)) in RBCs from IDA donors, and that there is a slight increase in the growth of P. falciparum in RBCs from IDA+Fe donors (22.8% (95% CI=2.7–46.7)) and RBCs from IR+Fe donors (18.9% (95% CI=5.0–33.9)); no difference was observed between P. falciparum growth in RBCs from IR+Fe donors and IDA+Fe donors ( Fig. 1e ). These data clearly indicate that IDA substantially attenuates the growth of P. falciparum parasites and that iron supplementation of donors with IDA reverses the protection provided by IDA against falciparum infection. Furthermore, these data suggest that iron supplementation of IR individuals may slightly increase propagation of erythrocytic stage P. falciparum. RBCs from donors with IDA are refractory to malaria infection Propagation of the erythrocytic stage of P. falciparum may be impeded at the point of (i) invasion, (ii) maturation or (iii) production of infectious daughter merozoites. To determine why P. falciparum infection of RBCs from IDA donors is reduced, we systematically assessed the capacity of P. falciparum to progress through each of these rate-limiting steps within RBCs from IDA donors compared with RBCs from IR donors. To assess invasion, we directly compare invasion of P. falciparum strains 3D7, Dd2 and FCR3-FMG into RBCs from IDA and IR donors with a barcoded RBC flow cytometry based invasion assay. To express the differential invasion of RBCs, we computed the susceptibility index (SI), which is the ratio of the relative risk of invasion of RBCs from IDA donors to that of RBCs from IR donors. An SI of 1.0 indicates no difference in parasite invasion between two RBC populations. In experiments with strains 3D7, Dd2 and FCR3-FMG, the mean SI of RBCs from IDA donors relative to RBCs from IR donors was 0.56 (95% CI=0.56–0.57), 0.52 (95% CI=0.52–0.53) and 0.70 (95% CI=0.69–0.71), respectively, indicating consistently reduced invasion of RBCs from IDA donors ( Fig. 2a ). We next assessed parasite maturation within RBCs from IDA donors by analysing Giemsa-stained thing blood smears, which were made every 6 h during the course of a 48-h intra-erythrocytic lifecycle. 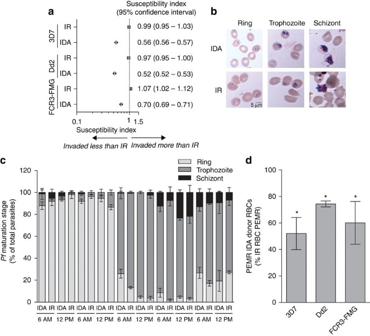Figure 2:P. falciparuminvasion and growth are reduced in RBCs from IDA donors. (a) Direct comparison of invasion into RBCs from either IDA or IR donors. Invasion experiments for RBCs from all IDA donors were performed independently and each experiment was performed in triplicate. Data show the mean SI of six independent experiments performed with RBCs from six IDA donors. The marker represents the SI point estimate and the bar represents the 95% CI. An SI of 1.0 indicates no difference in parasite invasion of the two RBC populations. (b,c) Comparison of the maturation ofP. falciparumin RBCs donated by IDA and IR donors. Geimsa-stained thin blood smears were made every 6 h and 1,000 RBCs were counted by light microscopy to determine the percent of pRBCs as well as parasite intra-erythrocytic stage of maturation. Data are from a representative experiment (with strain FCR3-FMG) of three independent experiments performed with RBCs from three IDA donors infected with eitherP. falciparumstrain 3D7, Dd2or FCR3. (b) Giemsa-stained thin blood smears ofP. falciparumring, trophozoite and schizont stage parasites in RBCs from an IDA and an IR donor. (c) Bars indicate percent frequency of parasite ring, trophozoite and schizont stages in RBCs from an IDA and IR donor at each 6 h time point. Error bars represent the s.d. (d) Comparison of the parasite erythrocyte multiplication rate (PEMR) ofP. falciparumwithin RBCs from IDA and IR donors. Bars represent PEMR ofP. falciparumin RBCs from IDA donors, normalized to the PEMR of parasites in RBCs from IR donors (% IR PEMR). Data are the mean of three independent experiments performed in triplicate with RBCs from three IDA donors. Error bars represent the s.d. Significance determined by two-tailed paired Student’st-test.*P<3E−6, compared with PEMR in RBCs from IR donors. We observed that parasites matured normally in iron-deficient RBCs, indicating that the reduced overall parasite growth in iron-deficient RBCs did not result from delayed maturation ( Fig 2b,c ). Finally, we measured the parasitized erythrocyte multiplication rate (PEMR) [17] , [18] of P. falciparum within RBCs from IDA donors as compared with RBCs from IR donors. For parasite strains 3D7, Dd2 and FCR3-FMG, RBCs from IDA donors (relative to RBCs from IR donors) had a reduced PEMR of 48.0% (s.d.±12.2), 25.7% (s.d.±2.2) and 39.9% (s.d.±9.3), respectively ( Fig. 2d ). In accordance with the PEMR data, we additionally observed fewer merozoites within IDA as compared with IR RBCs by microscopy (data not shown). Taken together, these data indicate that P. falciparum matures normally within RBCs from IDA donors, but that invasion into and production of infectious merozoites within RBCs from IDA donors are significantly reduced. These data additionally reveal that different P. falciparum isolates may exhibit different invasion and PEMR phenotypes in RBCs of IDA individuals. Figure 2: P. falciparum invasion and growth are reduced in RBCs from IDA donors. ( a ) Direct comparison of invasion into RBCs from either IDA or IR donors. Invasion experiments for RBCs from all IDA donors were performed independently and each experiment was performed in triplicate. Data show the mean SI of six independent experiments performed with RBCs from six IDA donors. The marker represents the SI point estimate and the bar represents the 95% CI. An SI of 1.0 indicates no difference in parasite invasion of the two RBC populations. ( b , c ) Comparison of the maturation of P. falciparum in RBCs donated by IDA and IR donors. Geimsa-stained thin blood smears were made every 6 h and 1,000 RBCs were counted by light microscopy to determine the percent of pRBCs as well as parasite intra-erythrocytic stage of maturation. Data are from a representative experiment (with strain FCR3-FMG) of three independent experiments performed with RBCs from three IDA donors infected with either P. falciparum strain 3D7, Dd2or FCR3. ( b ) Giemsa-stained thin blood smears of P. falciparum ring, trophozoite and schizont stage parasites in RBCs from an IDA and an IR donor. ( c ) Bars indicate percent frequency of parasite ring, trophozoite and schizont stages in RBCs from an IDA and IR donor at each 6 h time point. Error bars represent the s.d. ( d ) Comparison of the parasite erythrocyte multiplication rate (PEMR) of P. falciparum within RBCs from IDA and IR donors. Bars represent PEMR of P. falciparum in RBCs from IDA donors, normalized to the PEMR of parasites in RBCs from IR donors (% IR PEMR). Data are the mean of three independent experiments performed in triplicate with RBCs from three IDA donors. Error bars represent the s.d. Significance determined by two-tailed paired Student’s t -test. * P <3E −6 , compared with PEMR in RBCs from IR donors. Full size image Replacement of iron-deficient RBCs increases malaria growth The erythropoietic rate of iron-deficient individuals increases dramatically in response to iron supplementation, and elevated erythropoietic rate is hypothesized to increase an individual’s susceptibility to malaria [19] . As the iron biomarkers of individuals in the IDA+Fe group were indicative of an erythropoietic response to iron ( Table 1 ), we hypothesized that the replacement of iron-deficient RBCs with IR RBCs would explain the recovered growth of P. falciparum in RBCs from IDA+Fe donors ( Fig. 1 ). To determine whether the replacement of iron-deficient RBCs with young IR RBCs could explain the recovered growth of P. falciparum in RBCs donated by IDA+Fe individuals, we first compared P. falciparum infection of reticulocytes (CD71+) and mature RBCs (CD71−) from IDA + Fe donors. Consistent with P. falciparum’s reported preference for young RBCs, we observed 8.6% (s.d.±0.1) parasitization of reticulocytes (CD71+) and 4.5% (s.d.±0.4) parasitization of mature RBCs (CD71−) ( Fig. 3a ). However, (CD71+) reticulocytes accounted for only 1.6% (s.d.±0.9) of all RBCs and parasitized (CD71+) reticulocytes only contributed to 3.0% (s.d.±0.1) of the total number of parasitized RBCs ( Fig. 3b ). 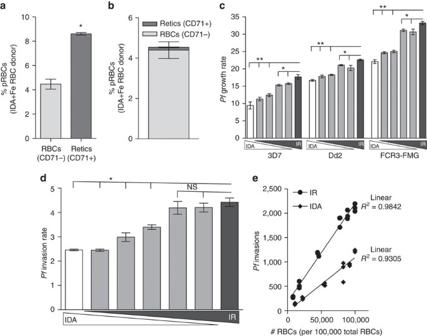Figure 3: Replacement of iron-deficient RBCs with iron-replete RBCs increasesP. falciparuminfection. (a,b)P. falciparum(strain 3D7) infection of reticulocytes (CD71+) and mature RBCs (CD71−) from an IDA+Fe donor. (a) Bars represent the percent of parasitized reticulocytes (CD71+) and mature RBCs (CD71−). Error bars represent the s.d. *P<0.0001. (b) Contribution of parasitized reticulocytes (CD71+) and parasitized mature RBCs (CD71−) to the total infection. Error bars represent the standard deviation. (c) Growth rate ofP. falciparumin RBC populations in which IDA RBCs were replaced with IR RBCs. RBCs were inoculated individually or together in the same wells at different ratios (100% IDA; 90% IDA and 10% IR; 75% IDA and 25% IR; 50% IDA and 50% IR; 25% IDA and 75% IR; 100% IR) and subsequently infected. Elongated triangles below thexaxis represent the percentage of IDA RBCs (white triangle) and IR RBCs (grey triangle) in the total RBC population. Bars represent parasite growth rates after one 96 h growth assay. Error bars represent the s.d. *P<0.01 and **P<0.0003. (dande) Invasion rate ofP. falciparuminto RBC populations in which IDA RBCs were replaced with IR RBCs. Differentially labelled RBC donors were inoculated individually or together in the same wells at different ratios (100% IDA; 90% IDA and 10% IR; 80% IDA and 20% IR; 50% IDA and 50% IR; 20% IDA and 80% IR; 10% IDA and 90% IR; 100% IR). Each invasion condition contained 20 × 106total RBCs. (d) Bars represent parasite invasion rate. Elongated triangles below thexaxis represent the percentage of IDA RBCs (white triangle) and IR RBCs (grey triangle) in the total RBC population. Error bars represent the s.d. *P<0.001, compared withP. falciparuminvasion rate into 100% IR RBCs. (e) Number of invasions events into IDA (diamonds) and IR (circles) RBCs as the frequency of each increases. Linear regression was used to determine the best fit lines for the data (IRR2=0.9842 and IDAR2=0.9305). Analysis of covariance was performed to compare the slopes of the lines and calculatedP<0.0001. The null hypothesis was no difference between the two RBC types (H0:βIron replete=βIron deficient,α=0.05) n.s., nonsignificant. Figure 3: Replacement of iron-deficient RBCs with iron-replete RBCs increases P. falciparum infection. ( a , b ) P. falciparum (strain 3D7) infection of reticulocytes (CD71+) and mature RBCs (CD71−) from an IDA+Fe donor. ( a ) Bars represent the percent of parasitized reticulocytes (CD71+) and mature RBCs (CD71−). Error bars represent the s.d. * P <0.0001. ( b ) Contribution of parasitized reticulocytes (CD71+) and parasitized mature RBCs (CD71−) to the total infection. Error bars represent the standard deviation. ( c ) Growth rate of P. falciparum in RBC populations in which IDA RBCs were replaced with IR RBCs. RBCs were inoculated individually or together in the same wells at different ratios (100% IDA; 90% IDA and 10% IR; 75% IDA and 25% IR; 50% IDA and 50% IR; 25% IDA and 75% IR; 100% IR) and subsequently infected. Elongated triangles below the x axis represent the percentage of IDA RBCs (white triangle) and IR RBCs (grey triangle) in the total RBC population. Bars represent parasite growth rates after one 96 h growth assay. Error bars represent the s.d. * P <0.01 and ** P <0.0003. ( d and e ) Invasion rate of P. falciparum into RBC populations in which IDA RBCs were replaced with IR RBCs. Differentially labelled RBC donors were inoculated individually or together in the same wells at different ratios (100% IDA; 90% IDA and 10% IR; 80% IDA and 20% IR; 50% IDA and 50% IR; 20% IDA and 80% IR; 10% IDA and 90% IR; 100% IR). Each invasion condition contained 20 × 10 6 total RBCs. ( d ) Bars represent parasite invasion rate. Elongated triangles below the x axis represent the percentage of IDA RBCs (white triangle) and IR RBCs (grey triangle) in the total RBC population. Error bars represent the s.d. * P <0.001, compared with P. falciparum invasion rate into 100% IR RBCs. ( e ) Number of invasions events into IDA (diamonds) and IR (circles) RBCs as the frequency of each increases. Linear regression was used to determine the best fit lines for the data (IR R 2 =0.9842 and IDA R 2 =0.9305). Analysis of covariance was performed to compare the slopes of the lines and calculated P <0.0001. The null hypothesis was no difference between the two RBC types (H 0 : β Iron replete = β Iron deficient , α =0.05) n.s., nonsignificant. Full size image Having clearly demonstrated that reticulocytes from IDA+Fe donors are more highly infected by P. falciparum , but that reticulocytes themselves only contribute marginally to the total infection, we next sought to definitively determine whether the replacement of iron-deficient with IR RBCs could explain the recovered growth of P. falciparum in RBCs from IDA+Fe donors. However, low incidence of IDA in our study setting, the difficulty of following iron-supplemented IDA individuals longitudinally through full recovery from iron deficiency, as well as the inability to use the common surrogates of RBC age (volume and density) against the background of changing host iron status, prevented us from studying the impact of an elevated erythropoietic rate on erythrocytic stage P. falciparum infection. Therefore, we modelled the effect of iron supplementation-mediated changes in RBC population dynamics on erythrocytic stage P. falciparum infection by assessing the impact of replacing RBCs from IDA donors with RBCs from IR donors on in vitro P. falciparum growth. Replacing 10, 25, 50 and 75% of the RBCs from IDA donors with RBCs from IR donors resulted in a steady increase in parasite growth rate; 75% replacement recovered 3D7, Dd2 and FCR3-FMG P. falciparum growth rate to 88.2% (s.d.±2.0), 89.7% (s.d.±2.5) and 92.3% (s.d.±1.1) that of the growth rate of in RBCs from IR donors, respectively ( Fig. 3c ). As the first step in the erythrocytic life cycle of the malaria parasite, erythrocyte invasion is a pivotal determinant of the magnitude of infection. Therefore, we utilized the barcoded RBC invasion assay to determine how iron-deficient and IR RBCs interact to shape P. falciparum invasion. Like growth rate, P. falciparum invasion rate increased as IDA RBCs were replaced with IR RBCs. Rate of invasion was fully recovered to IR levels once 80% of IDA RBCs were replaced with IR RBCs for all three parasite strains ( Fig. 3d and Supplementary Fig. 2a ). Furthermore, employment of the barcoded RBC invasion assay allowed for the full characterization of the kinetics of P. falciparum invasion into IDA and IR RBCs, as the frequency of each changed relative to the total RBC population. We observed that the number of P. falciparum FCR3-FMG invasions into IDA and IR RBCs increased linearly, as each RBC population increased in frequency, R 2 =0.984 and 0.931, respectively, and P. falciparum invasion as a function of IDA RBC abundance was significantly less than that of IR RBCs ( Fig. 3e ). Similar trends were observed for P. falciparum strains 3D7 and Dd2 ( Supplementary Fig. 2b and c ). Together, these results support the hypothesis that replacing an individual’s iron-deficient RBC population with IR RBCs would increase the host’s susceptibility to erythrocytic stage P. falciparum infection and clearly illustrate the impact RBC population dynamics have on potential parasite biomass and pathogenesis. Moreover, our use of the barcoded RBC invasion assay allowed for the definitive determination and characterization of the distribution of parasites in IDA and IR RBC populations, as the frequency of each changed. Effect of RBC population age structure on malaria infection Reticulocytes and young RBCs are preferentially invaded by P. falciparum [20] , [21] , and theoretical models predict that elevated reticulocytosis may increase the risk of high parasite density [19] , [22] . Because of the shortened lifespan of iron-deficient RBCs, there is a period in the course of an individual’s recovery from IDA at which point protective iron-deficient RBCs have been cleared from circulation and the remaining circulating RBCs are on average younger than that of an IR individual. To determine the capacity of young RBCs to shape P. falciparum infection, we (i) directly compare P. falciparum infection of young RBCs and RBCs of increasing age and (ii) model the effect of replacing young IR RBCs with old IR RBCs on P. falciparum growth and invasion in vitro . For these studies, we utilized two proxies for RBC age: RBC volume, which decreases with age [23] and is unaffected by ring stage parasitization [24] , and RBC density, which increases with increasing RBC age [23] . We observed that when RBCs from an IR donor were infected with P. falciparum , parasite infection increased with increasing RBC volume ( Fig. 4a ). To directly compare P. falciparum invasion of RBCs of different ages, we density separated RBCs from IR donors into four fractions of increasing RBC age: young, young adult, mature adult and old ( Supplementary Fig. 3A ). Decreasing MCV, reticulocyte content and Calcein fluorescence [25] confirmed the age separation of the RBCs ( Supplementary Fig. 3b–d ). We observed that the SI of young adult, mature adult and old RBCs to parasite invasion as compared with young RBCs was 0.85 (95% CI=0.82–0.90), 0.58 (95% CI=0.56–0.62) and 0.28 (95% CI=0.27–0.30), respectively ( Fig. 4b ). In accordance with previous reports [17] , [20] , [26] , young RBCs sustained a significantly greater growth rate than young adult, mature adult and old RBCs, with young RBCs supporting a growth rate 50% greater than old RBCs ( Supplementary Fig. 3e ), and compared with young RBCs the PEMR was reduced by 10% (s.d.±4.78), 15% (s.d.±1.16) and 19% (s.d.±2.23) in young adult, mature adult and old RBCs, respectively ( Supplementary Fig. 3f ). These data clearly demonstrate the preferential invasion of P. falciparum into young RBCs and show that the risk of RBCs to P. falciparum invasion relative to young RBCs decreases with increasing RBC age. All together we have confirmed (i) P. falciparum infection is more prevalent in young RBCs (ii) the increased capacity of young RBCs to support P. falciparum invasion and growth. 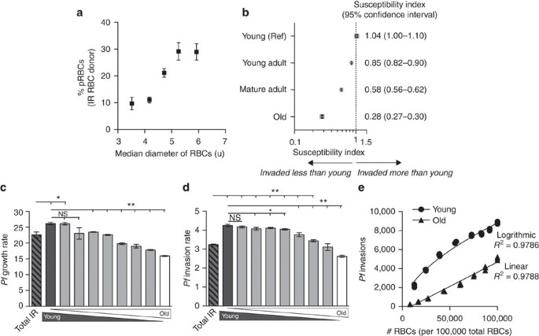Figure 4: The elevatedP. falciparuminfection supported by young RBCs is reversed as young RBCs are replaced with old RBCs. (a) PercentP. falciparum(strain 3D7) infection of RBCs of increasing diameter. Data points represent the % pRBCs of five gated RBC populations of increasing volume. Error bars represent the s.d. (b) Direct comparison ofP. falciparum(strain FCR3-FMG) invasion into RBCs of increasing age. IR RBCs were separated into five fractions of increasing density, a proxy for increasing RBC age (Supplementary Fig. 3a–d). The markers represent the SI point estimate and the bar represents the 95% CI. (c) Growth rate ofP. falciparum(strain FCR3-FMG) in RBC populations in which young IR RBCs were replaced with old IR RBCs (0%, 10%, 20%, 33%, 50%, 66%, 80%, 90% and 100% replacement young RBCs with old RBCs). Elongated triangles represent the percentage of young IR RBCs (gray triangle) and old IR RBCs (white triangle) in the total RBC population. Bars represent parasite growth rates after 96 h Error bars represent the s.d. *P<0.004 and **P<0.0003, compared to growth rate in 100% total IR and 100% young RBCs respectively. (dande) Invasion into RBC populations in which young IR RBCs were replaced with old IR RBCs. Differentially labelled young and old RBCs were inoculated individually or together in the same wells at different ratios (0%, 10%, 20%, 33%, 50%, 66%, 80%, 90% and 100% replacement young RBCs with old RBCs). (d) Bars represent invasion rates. Elongated triangles represent the percentage of young IR RBCs (gray triangle) and old IR RBCs (white triangle) in the total RBC population. Error bars represent the s.d. *P<0.05 and **P<0.003 (e) Number of invasions events into young (circles) and old (triangles) RBCs as the frequency of each increases. Linear regression was used to determine best fit lines. A linear function best fit old RBC data (R2=0.9788) and a logarithmic function best fit young RBC data (R2=0.9786). Analysis of covariance was performed to determine whether invasion data of old and young RBCs differed significantly,P<0.0001. The null hypothesis was no difference between the two RBC types (H0:βIron replete=βIron deficient,α=0.05) n.s., nonsignificant. Figure 4: The elevated P. falciparum infection supported by young RBCs is reversed as young RBCs are replaced with old RBCs. ( a ) Percent P. falciparum (strain 3D7) infection of RBCs of increasing diameter. Data points represent the % pRBCs of five gated RBC populations of increasing volume. Error bars represent the s.d. ( b ) Direct comparison of P. falciparum (strain FCR3-FMG) invasion into RBCs of increasing age. IR RBCs were separated into five fractions of increasing density, a proxy for increasing RBC age ( Supplementary Fig. 3a–d ). The markers represent the SI point estimate and the bar represents the 95% CI. ( c ) Growth rate of P. falciparum (strain FCR3-FMG) in RBC populations in which young IR RBCs were replaced with old IR RBCs (0%, 10%, 20%, 33%, 50%, 66%, 80%, 90% and 100% replacement young RBCs with old RBCs). Elongated triangles represent the percentage of young IR RBCs (gray triangle) and old IR RBCs (white triangle) in the total RBC population. Bars represent parasite growth rates after 96 h Error bars represent the s.d. * P <0.004 and ** P <0.0003, compared to growth rate in 100% total IR and 100% young RBCs respectively. ( d and e ) Invasion into RBC populations in which young IR RBCs were replaced with old IR RBCs. Differentially labelled young and old RBCs were inoculated individually or together in the same wells at different ratios (0%, 10%, 20%, 33%, 50%, 66%, 80%, 90% and 100% replacement young RBCs with old RBCs). ( d ) Bars represent invasion rates. Elongated triangles represent the percentage of young IR RBCs (gray triangle) and old IR RBCs (white triangle) in the total RBC population. Error bars represent the s.d. * P <0.05 and ** P <0.003 ( e ) Number of invasions events into young (circles) and old (triangles) RBCs as the frequency of each increases. Linear regression was used to determine best fit lines. A linear function best fit old RBC data ( R 2 =0.9788) and a logarithmic function best fit young RBC data ( R 2 =0.9786). Analysis of covariance was performed to determine whether invasion data of old and young RBCs differed significantly, P <0.0001. The null hypothesis was no difference between the two RBC types (H 0 : β Iron replete = β Iron deficient , α =0.05) n.s., nonsignificant. Full size image To determine the capacity of the age distribution of a RBC population to shape P. falciparum infection, we examined the effect of replacing young IR RBCs with old IR RBCs on P. falciparum growth in vitro . We observed 15.7% (s.d.±3.1) greater growth of P. falciparum in young IR RBCs as compared with density separated and then recombined (total) IR RBCs, and growth remained significantly greater when 10% of young RBCs were replaced with old RBCs. Following replacement of 33, 50, 66, 80 and 90% of young RBCs with old RBCs, P. falciparum growth rate steadily decreased ( Fig. 4c ). Consistent with P. falciparum growth, we observe that the rate of P. falciparum invasion into young RBCs is significantly greater than that of total IR RBCs (29.0% (s.d.±2.1)). Furthermore, we observed that as the frequency of young RBCs decreased from 100 to 50% and the frequency of old RBCs increased from 0 to 50%, the total rate of invasion decreased by only 4.9% (s.d.±0.7), maintaining a P. falciparum invasion rate significantly greater than that of the invasion rate of total RBCs. However, when the frequency of young RBCs fell from 50 to 0% and old RBCs increased from 50 to 100%, P. falciparum infection decreased steadily, ultimately falling by 45.7% (s.d.±1.9) ( Fig. 4d ). As young IR RBCs are at the greatest risk of P. falciparum invasion, we speculated that an insufficient merozoite inoculum might be responsible for the observed plateau in P. falciparum invasion. However, invasion experiments with double the inoculum of merozoites also resulted in a plateau in the rate of P. falciparum invasion when young RBCs accounted for more than 50% of the total RBCs population ( Supplementary Fig. 4a ). Moreover, the rate of P. falciparum invasion achieved with the higher inoculum was less than that of the lower inoculum invasion experiments ( Fig. 4d and Supplementary Fig. 4a ). We subsequently characterized the kinetics of P. falciparum invasion into young and old RBCs as the frequency of each changed relative to the total RBC population. We observed that like P. falciparum invasion of IDA and IR RBCs, the number of P. falciparum invasions into old IR RBCs increased linearly as old IR RBCs increased in frequency, R 2 =0.991. In contrast, the number of P. falciparum invasions into young IR RBCs as a function of young IR RBC abundance was best fit by a logarithmic function, R 2 =0.976 ( Fig. 4e ). The same kinetics of P. falciparum invasion were observed when experiments were performed with double the merozoite inoculum ( Supplementary Fig. 4b ). These results demonstrate that replacement of young IR RBCs with old IR RBCs reverses the elevated growth and invasion rate sustained by young IR RBCs. In addition, we show that the rate of P. falciparum invasion only begins to dramatically drop off once 50% of young IR RBCs have been replaced with old IR RBCs, and that this can be attributed to the logarithmic nature of P. falciparum invasion of young IR RBCs. Together, these data support the hypothesis that the effects of iron deficiency and iron supplementation on RBC physiology and erythropoietic rate are at least partially responsible for determining an individual’s risk of malaria infection ( Fig. 5 ). 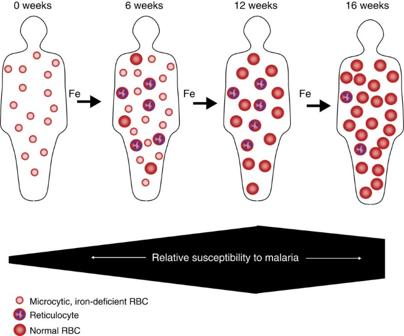Figure 5: Hypothesized impact of iron deficiency and iron supplementation on host RBC population dynamics and susceptibility to erythrocytic stage malaria infection. Recovery from IDA is a complex process, which varies between individuals. Iron supplementation of an individual with IDA (0 weeks) will result in reticulocytosis and the production of young iron-replete RBCs (6 weeks). 12 weeks after the initiation of supplementation, the majority of the iron-deficient RBCs, will have been cleared from circulation (iron-deficient and iron-replete RBCs have 90 and 120 day lifespans respectively). After 16 weeks of iron supplementation, iron status has been corrected and the age structure of the RBC population will be restored. As shown above, we hypothesize that individuals with IDA will be less susceptible to erythrocytic stage malaria. The induction of erythropoiesis in these individual by iron supplementation and subsequent replacement of the iron-deficient RBCs with young iron-replete RBCs will increase the susceptibility of the individual to erythrocytic stage malaria infection. The susceptibility to infection is predicted to peak at the point when all iron-deficient RBCs have been replaced, but the age distribution of iron-replete RBCs is on average younger than a fully recovered iron-replete individual. Finally, restoration of the normal distribution of RBC age will return an individual’s susceptibility to a normal level. Figure 5: Hypothesized impact of iron deficiency and iron supplementation on host RBC population dynamics and susceptibility to erythrocytic stage malaria infection. Recovery from IDA is a complex process, which varies between individuals. Iron supplementation of an individual with IDA (0 weeks) will result in reticulocytosis and the production of young iron-replete RBCs (6 weeks). 12 weeks after the initiation of supplementation, the majority of the iron-deficient RBCs, will have been cleared from circulation (iron-deficient and iron-replete RBCs have 90 and 120 day lifespans respectively). After 16 weeks of iron supplementation, iron status has been corrected and the age structure of the RBC population will be restored. As shown above, we hypothesize that individuals with IDA will be less susceptible to erythrocytic stage malaria. The induction of erythropoiesis in these individual by iron supplementation and subsequent replacement of the iron-deficient RBCs with young iron-replete RBCs will increase the susceptibility of the individual to erythrocytic stage malaria infection. The susceptibility to infection is predicted to peak at the point when all iron-deficient RBCs have been replaced, but the age distribution of iron-replete RBCs is on average younger than a fully recovered iron-replete individual. Finally, restoration of the normal distribution of RBC age will return an individual’s susceptibility to a normal level. Full size image Iron supplementation has clear nutritional benefits for children and pregnant women [2] , but iron is also an essential nutrient for most pathogens and as a result is a critical mediator of host–pathogen interactions [27] . Activation of the host innate immune system by the malaria parasite or other infectious organisms triggers reduction in iron absorption, redistribution of existing iron stores and decreases erythropoiesis, which effectively limits the availability of iron to invading pathogens. It is unknown what host iron (mosquito or human) P. falciparum is able to access and utilize nor how the parasite circumvents the host’s attempt to restrict iron. It has been previously postulated that as occurs with other pathogens [28] , iron deficiency inhibits P. falciparum infection via iron deprivation. Although the malaria parasite may find iron less readily available in an iron-deficient host, our work reveals an alternate cellular mechanism by which iron deficiency may protect against malaria. Our study of the relationship between iron deficiency, iron supplementation and erythrocytic stage P. falciparum infection highlights how by altering the dynamics of the human hosts RBC population iron deficiency and iron supplementation shape erythrocytic stage P. falciparum infection. Clinical studies in different field sites have reported that iron deficiency correlates with protection from malaria. In Malawian children, baseline iron deficiency was associated with significant reductions in the subsequent risks of both parasitemia (45%) and malaria (51%) [29] . Similarly, in Tanzanian children, baseline iron deficiency significantly decreased the odds of subsequent parasitemia (23%) and severe malaria (38%) [6] . In addition, in two studies of pregnant women, iron deficiency was associated with a decreased prevalence of placental malaria, a major cause of neonatal and maternal morbidity [3] , [4] . Our results—that iron-deficient RBCs impair parasite propagation in vitro ( Fig. 1 )—are consistent with these clinical findings, and provide valuable insight into a cellular mechanism for the observations made in the clinical setting. In our study of P. falciparum growth in RBCs from IDA donors, we reveal that RBCs from IDA donors are refractory to P. falciparum invasion and support a lower PEMR but that parasite maturation is normal ( Fig. 2 ). There are multiple physiological differences between iron-deficient and IR RBCs that may contribute to the impaired invasion into and replication within iron-deficient RBCs. These include greater osmotic fragility and membrane rigidity, accelerated ageing in vivo [30] , [31] , [32] , [33] , lower Hgb content and smaller size (microcytosis). Iron supplementation has long been hypothesized to increase malaria risk, and this issue has garnered recent attention after a large-scale nutritional supplementation study in Tanzanian children was halted owing to significantly increased mortality among those receiving iron [8] . Although it remains unclear whether the increased mortality rate was secondary to malaria, this potential for harm has complicated recommendations for widespread supplementation and has caused iron supplementation programmes in malaria endemic countries to be suspended. In a more recent randomized trial of Tanzanian children, iron supplementation increased the risk of malaria by 41% in iron-deficient but not in IR children [8] . Notably, our studies are consistent with the Tanzania study. Specifically, we observed increased parasite growth in RBCs donated by iron-supplemented IDA individuals and a modest effect in RBCs donated by iron-supplemented IR individuals ( Fig. 1 ). As individuals in the iron-supplemented IDA group were observed to be undergoing an erythropoietic response to iron supplementation ( Table 1 ), we proceeded to investigate the effect of replacing iron-deficient RBCs with IR RBCs and young RBCs with old RBCs on P. falciparum erythrocyte infection. We demonstrate that P. falciparum growth and invasion rates increase when iron-deficient RBCs are replaced with IR RBCs ( Fig. 3 ). Furthermore, we show that young RBCs support greater P. falciparum growth and invasion rates than total IR RBCs and that the replacement of young RBCs with old RBCs reverses the effect of young RBCs on parasite growth and invasion ( Fig. 4 ). Finally, in the course of these experiments, our use of barcoded RBC flow cytometry invasion assay has provided novel insight into the relationship between the frequency of a RBC subset in the total RBC population and P. falciparum infection ( Figs 3e and 4e ). In summary, our results demonstrate that the changes in the RBC population that occur during recovery from IDA enhance parasite propagation. It should be noted that our work exclusively focuses on the influence of iron deficiency and iron supplementation on the susceptibility of the human host’s RBC to malaria infection, and does not address the potential effect of serum iron [13] or additional factors, which may function in vivo , including growth of the hepatic stage of the parasite [34] , rosetting and cytoadherence to the endothelium, accelerated clearance of parasitized RBCs [35] , [36] , effects of innate immune factors such as hepcidin [11] and lipocalin 2 (ref. 37 ), or adaptive immune function. We have previously reported that both transferrin and ferric citrate increase the bioavailable iron pool of trophozoite-infected RBCs but not that of uninfected RBCs [13] . It is possible that parasite growth may be enhanced by the transient increase in serum iron that is observed in IR individuals who are given oral iron supplementation [12] . Further investigations need to be conducted to explore the extent to which iron deficiency and iron supplementation shape other aspects of malaria pathogenesis. Our findings, taken together with those from field studies, raise the important medical and public health question: How can iron supplementation be safely administered to IDA children in malarious areas? A critical implication of these observations is that reconstitution of red cell mass in anaemic patients would be expected to transiently enhance susceptibility to malaria ( Fig. 5 ), which may inform the on-going debate as to whether fortification with iron would be safer than supplemental iron. Our data implies that, where P. falciparum is endemic, treatment of anaemia with iron supplementation should be accompanied by malaria preventive measures, such as malaria prophylaxis, bed nets and increased active surveillance and access to health care. Additional questions raised by this study are: Does iron deficiency in African children represent an evolutionarily advantageous phenotype that derives from polymorphisms in iron homeostasis? What molecular mechanisms confer protection from malaria in the setting of microcytosis, and can these protective mechanisms be exploited by medical interventions? Future clinical and translational studies will be needed in order to design safe and effective interventions to address the twin burdens of iron deficiency and falciparum malaria. Clinical Study participants included healthy, HIV-negative, non-pregnant donors over 18 years of age with and without IDA. Exclusion criteria included: on-going inflammation or infection, previous history of malaria, travel to malaria endemic areas, malignancy, sickle cell disease (or trait), thalassemia (or trait for either thalassemia-α or -β). This study was approved by the University of North Carolina Institutional Review Board, Protocol # 09-0559, and informed consent was obtained from all subjects. Study participants with Hgb >11 g dl −1 and ferritin >12 ng ml −1 were classified as IR and participants with Hgb <11 g dl −1 and ferritin <12 ng ml −1 were classified as IDA. IDA+Fe donors were identified by their personal physicians for participation in our study. Subjects were included in the IDA+Fe group if they fit the criteria for IDA and had been prescribed high-dose oral ferrous sulfate, 60 mg (9–12.6 mg kg −1 ) elemental iron orally three times per day or intravenous iron at a dosage determined by their personal physician using the following equation: Dose=0.0442 [desired Hgb−observed Hgb] × LBW+[0.26 × LBW]. Healthy donors took 325 mg of ferrous sulfate once daily for the 2-month duration of the study. These donors donated 40 ml of blood on three occasions— at enrollment and two subsequent monthly intervals. An additional group of healthy donors served as the IR control group. Non-anaemic donors with low-iron stores (Hgb >11 g dl −1 , ferritin <12 ng ml −1 ) were excluded. Full iron panels were obtained for each study participant and mean values for each group are reported in Table 1 . Parasite culture P. falciparum parasite strains 3D7, Dd2 and FCR3-FMG were cultured in RBCs from O+, IR donors at 2–3% haematocrit and Albumax Complete Media (ACM)–RPMI 1640 (Sigma-Aldrich) with 10% AlbuMAX II (Gibco), 1 mM hypoxanthine (Sigma-Aldrich), 20 mM L -glutamine (Cellgro), 0.45% glucose (Cellgro) and 0.01 ng ml −1 gentamicin (Sigma-Aldrich). AlbuMAX II was used to supplement the media in place of human serum to isolate the effects of the RBCs from different experimental groups. All RBCs used for parasite culture were obtained from well-characterized IR O+ donors and used within 14 days of being drawn. Cultured parasites were maintained between 0.5 and 10% at 37 °C, in an atmosphere of 5% O 2 , 5% CO 2 and 90% N 2 with continuous shaking. Early ring stage parasites were synchronized with 5% (w/v) D -sorbitol. Synchronization was repeated at 20 and 40 h to achieve a tightly synchronized parasite population. Growth assay P. falciparum parasites from routine cultures were seeded as rings at 0.5% initial parasitemia in 1% haematocrit in ACM in triplicate in 96-well plates. Parasites were maintained for 96 h under standard culture conditions and the media was changed daily. At 96 h, parasite cultures were split back to 0.5% parasitemia and maintained as described for an additional 96 h ( Supplementary Fig. 1 ). Parasites were stained at all 0 and 96 h time points with 1 × DNA dye SYBR Green I (Invitrogen) as described in ref. 38 , and fixed in 1% paraformaldehyde and 0.0075% glutaraldehyde (Electron Microscopy Sciences) in Alsever’s Solution (Sigma-Aldrich) for 30 min at 4 °C. Fixative was removed and cells were stored in PBS at 4 °C until analysis by flow cytometry. Growth rate reflects the fold increase in RBC parasitization between 0 and 96 h. To identify parasitized reticulocytes, cultures were stained with 0.5 μM DNA dye SYTO 61 (Invitrogen) [13] , [39] and PE-conjugated mouse anti-human CD71 antibody (Miltenyi Biotech) and analysed by flow cytometry. Barcoded RBC invasion assay RBCs were labelled with 5 μM of either CellTrace Violet or CellTrace Far Red DDAO-SE (Invitrogen) as described [39] . Violet- and DDAO-labelled RBCs were combined in ACM and delivered in triplicate into 96-well plates and subsequently seeded with schizonts to achieve 1.5–2% parasitized RBCs. Parasites were maintained for 12–18 h under standard culture conditions to allow for schizont rupture and subsequent invasion of CellTrace-labelled RBCs. The invasion of P. falciparum into Violet- and DDAO-labelled RBCs was directly compared by measuring the SI, defined as the ratio of the prevalences of infected Violet RBCs to infected DDAO RBCs [40] . Note that the SI is different from the previously described selectivity index [18] , [41] . The selectivity index has been used to report the number of multiply infected cells, whereas the SI defines the relative susceptibility to invasion of two different types of RBCs. Parasite erythrocyte multiplication rate assay Trophozoite-infected cultures were magnetic activated cell sorting (MACS) purified and seeded into experimental RBCs to achieve 1.5–2% pRBCs and incubated for 48 h to allow for invasion of merozoites into experimental RBCs and their subsequent development into trophozoites inside the experimental RBCs. Experimental RBC parasite density was determined and the same number of infected experimental RBCs was seeded into separate wells containing target RBCs (from an IR donor) to achieve 1.5–2% pRBCs. Cultures were then incubated for 12–18 h to allow merozoites produced within experimental RBCs to invade target RBCs, allowing for assessment of the PEMR [17] , [18] . Following invasion of target RBCs, cells were stained with SYBR Green I and analysed by flow cytometry to determine the total number of ring pRBCs. PEMR reflects the number of merozoite invasions of target RBCs per schizont infected experimental RBC. Density separation RBCs were separated into five fractions with a modified version of previously described density gradient centrifugation method [23] . Briefly, blood was collected into acid citrate dextrose and plasma was subsequently removed by centrifugation for 15 min at 800 g . Packed cells were resuspended at 50% haematocrit in RPMI, and passed over a 2:1 (w/w) α-cellulose/microcrystalline cellulose column to remove lymphocytes [42] . Following lymphocyte depletion, RBCs were washed twice with RBC buffer (10 mM HEPES, 12 mM NaCl, 115 mM KCl, 5% BSA). RBCs were layered onto a 65, 60, 55 and 50% discontinuous Percoll gradient and then centrifuged for 25 min at 1,075 g . Each of the five fractions was removed, washed twice with RBC buffer and stored at 4 °C for up to 5 days. Decreasing MCV, reticulocyte content and Calcein fluorescence [25] of the five fractions confirmed the age separation of RBCs ( Supplementary Fig. 3c–g ). For barcoded RBC invasion assays and growth assays, which utilized density separated RBCs, recombined RBCs were included as a ‘total’ RBC control. Flow cytometry Growth, invasion and infectious merozoite production assays were analysed by flow cytometry using either a modified FACS-Calibur with two lasers 30 mW 488 Diode Pumped Solid State laser and a 25-mW 637 red diode laser (FACS-Calibur; Becton Dickinson, modified by Cytek Development) or a Beckman-Coulter (Dako) CyAn ADP. Channels and probes used on the FACS-Calibur included: SYTO 61 (637 nM, 666/27 bandpass), PE (488 nM, 585/42 bandpass) and SYBR Green I (488 nM, 530/30 bandpass). FACS-Calibur data were collected using FlowJo CE and analysed with Summit v5.1. Channels and probes used on the Dako cyan included: CellTrace Violet (405 nM, 450/50 bandpass), SYBR Green I (488 nM, 530/40 bandpass) and CellTrace DDAO-SE (635 nM, 665/20 bandpass). Data from the Cyan cyotometer were collected and analysed with Summit v4.3.01. Linear amplification of forward scatter was used to set event threshold in order to exclude cell debris, microparticles and doublets. Electronic volume of uninfected RBCs and pRBCs was assessed on a Beckman Coulter Cell lab Quanta (Beckman Coulter). Channels and probes used on the Quanta included: SYBR Green I (488 nM, 525/40 bandpass). National Institute of Standards and Technologies-certified beads standard L2 2 μm, L5 5 μm and L10 10 μm (Beckman Coulter) were used to calibrate electronic volume. Calibrated data were expressed as both electronic volume (μm 3 ) and diameter (μm). Quanta data were collected with Cell Lab Quanta Collection Software for Instrument Control and analysed with Kaluza (Beckman Coulter). For all experiments, samples were diluted to 0.001–0.002% haematocrit and 100,000–500,000 total events were collected. Statistical methods All experiments were performed in triplicate. Results are from either one representative experiment or the combined results of at least three independent experiments. Parasite growth rate and infectious merozoite production experiments were analysed with two-tailed Student’s t -test and one-way analysis of variance (GraphPad Prism 5). Data from all in vitro growth studies were pooled and analysed using random effects regression ( Fig. 1d,e ). The dependent variable in the analysis was the logarithm of the ratio of the percent pRBCs at 96 h (final) and 0 h (initial). In addition, to the usual variation independently affecting each observation, we fitted two higher levels of variance: variation between individuals and day-to-day variation in parasite ‘preparations’ taking account of the fact that in this data set these two variance components were cross (rather than the more usually encountered nested design). We fitted two exposure variables, iron status and iron supplementation, both as binary variables, and their interaction, focusing on three contrasts: supplemented IDA versus supplemented IR donors; supplemented versus non-supplemented IDA donors; supplemented versus non-supplemented IR donors. All experiments were performed in triplicate with three P. falciparum strains (3D7, Dd2 and FCR3-FMG) and consisted of three serial 96 h growth assays ( Supplementary Fig. 1 ); P. falciparum strain, growth assay number and their (highly significant) interaction were fitted as binary covariates. We noted that when 0 h (initial) percent pRBCs was greater than 1, the second growth assay always gave anomalous low results (most likely due to a saturation effect). As these data were uninformative and yet added noise to the analysis, we omitted all such cases while noting that although their inclusion increased the standard errors, it did not change the same general conclusions of the analysis. This model was fitted using Stata’s xtmixed procedure (v12, Stata Corp). To compare the susceptibility of different RBC types to invasion by P. falciparum , an unadjusted odds ratio was used to calculate the SI. All statistical analyses for invasion experiments were performed with Stata/IC (v10, Stata Corp). Linear regression was employed to investigate the associations between host iron status and parasite invasion in vitro using percent of RBCs from IDA or IR donors as the independent variable and total invasions/1 × 10 5 RBCs as the dependent variable ( Fig. 3e ). Analysis of covariance was conducted to determine whether the invasion into the two groups were the same. An α of 0.05 was set a priori to determine statistically significant differences. Similar analysis was done to better understand associations between RBC age and parasite invasion ( Fig. 4e ). How to cite this article: Clark, M. A. et al . Host iron status and iron supplementation mediate susceptibility to erythrocytic stage Plasmodium falciparum . Nat. Commun. 5:4446 doi: 10.1038/ncomms5446 (2014).